Conventional tree height–diameter relationships significantly overestimate aboveground carbon stocks in the Central Congo Basin Policies to reduce emissions from deforestation and forest degradation largely depend on accurate estimates of tropical forest carbon stocks. Here we present the first field-based carbon stock data for the Central Congo Basin in Yangambi, Democratic Republic of Congo. We find an average aboveground carbon stock of 162±20 Mg C ha −1 for intact old-growth forest, which is significantly lower than stocks recorded in the outer regions of the Congo Basin. The best available tree height–diameter relationships derived for Central Africa do not render accurate canopy height estimates for our study area. Aboveground carbon stocks would be overestimated by 24% if these inaccurate relationships were used. The studied forests have a lower stature compared with forests in the outer regions of the basin, which confirms remotely sensed patterns. Additionally, we find an average soil carbon stock of 111±24 Mg C ha −1 , slightly influenced by the current land-use change. Tropical forests represent a crucial carbon pool as they, reportedly, store 40–50% of all terrestrial carbon [1] , [2] and influence the global carbon balance when changes are induced due to climate change [3] and anthropogenic disturbances. In order to understand and quantify tropical forest carbon uptake and losses, accurate carbon stock reference data are needed [4] , as well as estimates of carbon fluxes resulting from both natural processes and land-use changes [1] , [5] . The accuracy of these reference data is essential for the implementation of climate mitigation policies to reduce emissions resulting from deforestation and forest degradation (REDD, UN Framework Convention on Climate Change, www.un-redd.org ) [6] , [7] . Currently, the uncertainty associated with these data is high and there are still large gaps in our knowledge with respect to the actual amount of carbon stored in tropical forests and the stability of this pool [4] . In African tropical forests, in particular, there are major challenges with respect to estimating carbon stocks and fluxes. Saatchi et al. [8] developed a benchmark map of carbon stocks across the tropics, predicting a gradient in Central Africa with highest stocks in western and eastern parts of the Congo Basin. This gradient is not always predicted [9] , and more data is needed for effective mapping, which is dependent on spatially extensive ground-based measurements to reduce regional uncertainties. To date, African tropical forests have been underrepresented in carbon research mainly due to a lack of resources for scientific research, limited logistical support, poor infrastructure and periodic political instability [9] , [10] . Only a limited number of inventoried and permanent monitoring plots have been established given the considerable extent of the African tropical forest [11] . The few available inventoried plots are unevenly distributed, with a high concentration in the outer regions of the Congo Basin, leaving the centre of the basin unexplored [10] , [11] . Biomass estimates for these plots have been extrapolated to the entire African tropical forest based on pan-tropical allometric equations [12] , [13] . These equations are generally parameterized without data from the African continent due to the lack thereof [13] . Only the study by Feldpausch et al. [14] has recently expanded the frequently used pan-tropical Chave et al. [13] equation with African data from the western Congo Basin. The robustness and accuracy of this equation has been noted for some African regions [15] , [16] , with its strength lying in the large sample size of tropical trees compared with the other equations. Nevertheless, the use of pan-tropical equations [12] , [13] in unstudied areas needs to be done with care as it could produce systematic errors in carbon stock estimates, specifically if not all variables, namely diameter, wood density and tree height, are accounted for. Here we report the first inventory-based carbon data obtained from a central location in the Congo Basin, situated in the UNESCO Man and Biosphere (MAB) reserve at Yangambi (YGB), Democratic Republic of Congo (DRC) ( Fig. 1 ), with estimates for both aboveground live tree and soil carbon stocks. Thirteen 1-ha plots are established in intact old-growth forest, including two forest types namely, mixed semideciduous ( n =8) and riparian mono-dominant evergreen Gilbertiodendron dewevrei ( n =5) forests. In the mixed forests, the species Scorodophloeus zenkeri , Panda oleosa , Anonidium mannii , Petersianthus macrocarpus , Staudtia kamerunensis and Erythrophleum suaveolens are abundant. In addition, to assess the effect of deforestation and regrowth at local scales, seven plots of 1 ha are established in previously deforested areas of mixed semideciduous forests, with varying regrowth ages after slash-and-burn agriculture, namely fallow ( n =3) next to young ( n =3) and old ( n =1) regrowth forest. Soil carbon stocks to a depth of 100 cm are quantified for all forest types except for the old regrowth forest. A comparison of aboveground carbon stocks in old-growth forests is made with AfriTRON sites [11] in western and eastern Congo Basin, in order to assess whether our first ground-based observations for this important region confirm the spatial trends observed by remote sensing [8] , [9] and to quantify possible intrinsic differences in carbon stocks. 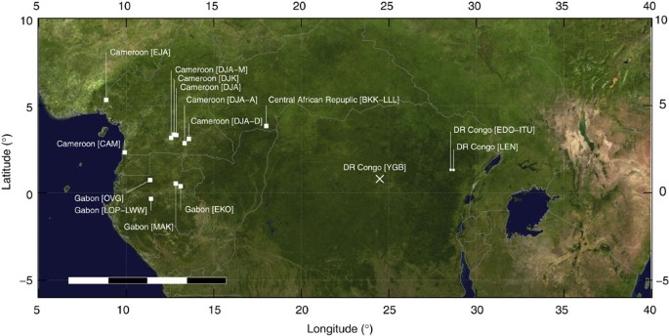Figure 1: Site locations. MODIS composite (NASA, Blue Marble) with the YGB study site and AfriTRON sites superimposed11. The sites are separated into different regions: squares indicate western Congo Basin sites, circles indicate eastern Congo Basin sites, and the cross indicates the Central Congo Basin site in YGB. In the scale bar, one block equals 250 km. Figure 1: Site locations. MODIS composite (NASA, Blue Marble) with the YGB study site and AfriTRON sites superimposed [11] . The sites are separated into different regions: squares indicate western Congo Basin sites, circles indicate eastern Congo Basin sites, and the cross indicates the Central Congo Basin site in YGB. In the scale bar, one block equals 250 km. Full size image YGB aboveground carbon stocks are lower With an aboveground carbon stock in live free-standing woody stems (minimum diameter 10 cm) in old-growth forest at YGB of 162±20 Mg C ha −1 , our estimates are 19% lower and significantly different ( P <0.001, Df=2) from estimates at the AfriTRON sites [11] ( Fig. 2 ) in the Congo Basin. Lewis et al. [11] report an average of 202 Mg C ha −1 for African tropical forest, and an even higher average in the Congo Basin, with 243 Mg C ha −1 for the western Congo Basin and 259 Mg C ha −1 for eastern Congo Basin sites ( Figs 1 and 2 ). Although the AfriTRON data show a large degree of variability within each geographic region, most AfriTRON sites have a significantly higher carbon stock than those estimated for YGB ( Fig. 2 ). The lower aboveground carbon stock at YGB is very remarkable and can be attributed to a different forest structure, where trees do not reach the same height for a given tree diameter as in the western or eastern Congo Basin ( Fig. 3 ). When comparing tree height–diameter regression curves developed for Central Africa [11] , [14] , [17] with those based on the YGB dataset, we found an asymptotic height difference of 9.4±0.9 m ( Fig. 3 , Table 1 ) resulting in an overestimation in aboveground carbon stocks of 12–25% (median 24%) equivalent to 29–62 Mg C ha −1 (median 53 Mg C ha −1 ). This results in an overestimated mean carbon stock of 212±24 Mg C ha −1 ( Fig. 2 , red points). This is a first indication that height–diameter allometry in some regions in Central Africa can differ from general regressions for Central Africa [14] , [17] , and that more localized height–diameter allometry is required. 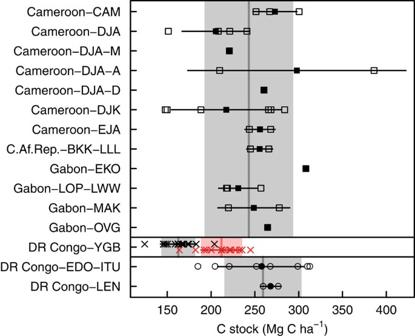Figure 2: Comparison between aboveground carbon stock at YGB and sites from the AfriTRON network. Sites from the AfriTRON network11are grouped according to location, West Congo Basin (squares) and East Congo Basin (circles), respectively. All acronyms refer to the applied site names in the AfriTRON network. Aboveground carbon stocks at YGB are incorporated as a separate region, Central Congo Basin (crosses). All carbon stocks are based on the same allometric equation for biomass13. For the YGB site, a distinction is made between carbon stocks estimated using a site-specific height–diameter relationship (grey line indicates mean) and a height–diameter relationship proposed for Central Congo Basin14(red line indicates mean). The overall mean carbon stocks for the separate regions—West Congo Basin, Central Congo Basin and East Congo Basin—are indicated by a grey line. The grey and red boxes indicate s.d. values along the mean. The significantly lower carbon stocks at YGB are emphasized, and the possible overestimation using the generalized height–diameter relationship for Central Congo Basin by Feldpauschet al.14is indicated in red. Within each region, a detailed representation of the same data grouped into clusters with plot locations close together11is shown indicating the large heterogeneity associated with carbon stock estimates, with all individual plot estimates (open symbols) and the mean of the cluster (filled symbols) including s.d. Figure 2: Comparison between aboveground carbon stock at YGB and sites from the AfriTRON network. Sites from the AfriTRON network [11] are grouped according to location, West Congo Basin (squares) and East Congo Basin (circles), respectively. All acronyms refer to the applied site names in the AfriTRON network. Aboveground carbon stocks at YGB are incorporated as a separate region, Central Congo Basin (crosses). All carbon stocks are based on the same allometric equation for biomass [13] . For the YGB site, a distinction is made between carbon stocks estimated using a site-specific height–diameter relationship (grey line indicates mean) and a height–diameter relationship proposed for Central Congo Basin [14] (red line indicates mean). The overall mean carbon stocks for the separate regions—West Congo Basin, Central Congo Basin and East Congo Basin—are indicated by a grey line. The grey and red boxes indicate s.d. values along the mean. The significantly lower carbon stocks at YGB are emphasized, and the possible overestimation using the generalized height–diameter relationship for Central Congo Basin by Feldpausch et al. [14] is indicated in red. Within each region, a detailed representation of the same data grouped into clusters with plot locations close together [11] is shown indicating the large heterogeneity associated with carbon stock estimates, with all individual plot estimates (open symbols) and the mean of the cluster (filled symbols) including s.d. 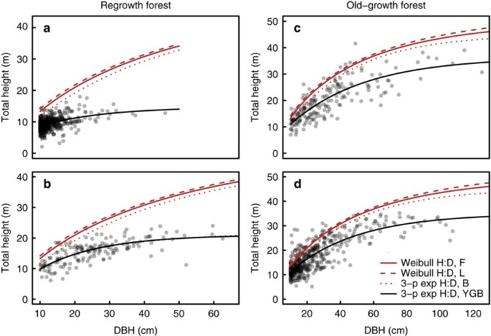Figure 3: Height–diameter models for different inventoried forest types at the YGB reserve in the Central Congo Basin. Comparison is made between regrowth and old-growth forests using different scales. (a) Fallow; (b) Young regrowth forest; (c) mixed old-growth forest; (d) mono-dominant old-growth forest. In black: the three-parameter exponential height–diameter (H:D) model optimized for the YGB site. In red: regional models for Central Africa. Weibull H:D, F, Feldpauschet al.14model; Weibull H:D, L, model used by Lewiset al.11(dashed); 3-p exp H:D, B, Baninet al.17model (dotted). The use of regional models results in an overestimate of tree heights and the biomass estimates are thus affected. Full size image Figure 3: Height–diameter models for different inventoried forest types at the YGB reserve in the Central Congo Basin. Comparison is made between regrowth and old-growth forests using different scales. ( a ) Fallow; ( b ) Young regrowth forest; ( c ) mixed old-growth forest; ( d ) mono-dominant old-growth forest. In black: the three-parameter exponential height–diameter (H:D) model optimized for the YGB site. In red: regional models for Central Africa. Weibull H:D, F, Feldpausch et al. [14] model; Weibull H:D, L, model used by Lewis et al. [11] (dashed); 3-p exp H:D, B, Banin et al. [17] model (dotted). The use of regional models results in an overestimate of tree heights and the biomass estimates are thus affected. Full size image Table 1 Coefficients for height–diameter relationship in a three-parameter exponential regression model. Full size table Tree height is the determining structural factor To explore in more detail the forest structural parameter responsible for the observed lower aboveground carbon stocks, we compared our data in more detail with datasets from sites in the Dja Faunal Reserve in Cameroon in the west of the Congo Basin and in the Ituri Dynamics Plots in the east, with a distinction of mixed and mono-dominant G. dewevrei forest types ( Table 2 ). For these areas, carbon stocks, basal area, stem density and wood density were available from literature, but explicit height data are lacking. In addition, data on soil and climate are available. By comparing mixed and mono-dominant plots separately, we were able to get a better view on the structural parameters driving the biomass differences. Table 2 Aboveground carbon stock in relation to structural and climate parameters for study sites. Full size table For mixed forests in these three sites, aboveground carbon stocks do not follow the same spatial gradient as generally seen for the Congo Basin [8] , with the Dja mixed forests showing smaller stocks, similar to the YGB ones. In the Dja reserve, a lower ( P <0.03) basal area is found, whereas both stem density and wood density are not significantly different from that in the YGB mixed forest ( P =1). The combination of a lower basal area with the same amount of trees in the plots in Dja, indicates that the average tree diameter is lower than that in YGB. In order to reach a similar carbon stock as in YGB, for a specific diameter, trees need to grow taller. This shows that differences in height–diameter relationships are a driver for the amount of carbon stored in these sites. Mixed forests in Ituri represent a significantly ( P =0.01) larger carbon stock than in YGB. Comparison of the structural parameters shows that a higher mean wood density ( P <0.001) is found in Ituri than in YGB with other variables ( Table 2 ) statistically indistinguishable ( P >0.6). This shows that the species composition is an important factor determining the larger carbon stock in Ituri, with a tendency for species with a higher wood density. This does not preclude that additional differences in height–diameter relationships could be present. In the mixed forests of these two regions, both basal area and stem density are similar. This indicates that the average tree diameter in both regions is similar and that a different maximal tree height attained in these forests could be the driver for the difference in carbon stock. By considering the mono-dominant G. dewevrei forests for the three regions, we exclude the influence of species composition on carbon stock. A significantly lower ( P <0.001) carbon stock is found in YGB, whereas all other forest stand variables are similar ( Table 2 ). The basal area in YGB is slightly lower ( P =0.04) than in Ituri, but similar to the values in Dja. With stem density being not significantly different for all regions, this indicates that mono-dominant forests in YGB do not have a lack of trees with a large diameter compared with the other regions. Mean wood density is slightly lower in YGB, although not significantly ( P =0.1). Consequently, the remaining determinative variable for the estimation of carbon stock is the total tree height reached in these mono-dominant forests, which clearly confirms our overall conclusion that tree height is largely explaining the significantly lower stock in YGB. Land-use change effect on above- and belowground carbon stock We estimated that aboveground carbon stocks in live trees with a minimum diameter of 10 cm in intact old-growth forest average 162±20 Mg C ha −1 , with no significant differences between the different old-growth forest types examined ( Fig. 4 ). For previously deforested plots, a lower aboveground carbon stock is found, varying according to land-use type and the age of any regenerated forest patch, with higher values for older plots with forest regrowth. There is, however, no corresponding difference in soil carbon stocks between intact and degraded forest plots. Soil carbon stocks to a depth of 100 cm in intact forest averaged 111±24 Mg C ha −1 and was equivalent to 68% of the aboveground stock. A significantly higher stock is found in mono-dominant forests with an average of 128±27 Mg C ha −1 , compared with 95±11 Mg C ha −1 in mixed forests ( Fig. 4 ). Even after forest clearing of mixed forest sites, the soil carbon stock remains high, although a gentle gradient is observable. Soil carbon stocks in fallow plots average 74±8 Mg C ha −1 and increase significantly with regrowth age as young regrowth forest shows an average of 101±22 Mg C ha −1 and thus return to the amount of soil carbon stock of the mixed forest from which they originate ( Supplementary Table S1 ). 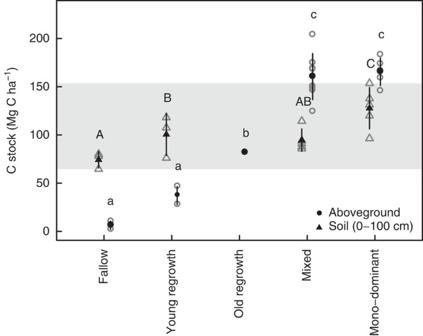Figure 4: Aboveground and soil carbon stock per forest type for inventory plots in the YGB reserve. Forest types are arranged from degraded to old-growth forest and show the impact of deforestation on aboveground carbon stock (circles) and soil carbon stock (triangles). The grey box indicates the variability range for soil carbon stocks. Significance from Fisher’s least significance difference test is visualized, with uppercase letters for the soil carbon stock and lowercase letters for the aboveground carbon stock. Values not sharing a common letter differ significantly. Figure 4: Aboveground and soil carbon stock per forest type for inventory plots in the YGB reserve. Forest types are arranged from degraded to old-growth forest and show the impact of deforestation on aboveground carbon stock (circles) and soil carbon stock (triangles). The grey box indicates the variability range for soil carbon stocks. Significance from Fisher’s least significance difference test is visualized, with uppercase letters for the soil carbon stock and lowercase letters for the aboveground carbon stock. Values not sharing a common letter differ significantly. Full size image Our observations, of lower aboveground carbon stocks for the Central Congo Basin, confirm patterns found by remote sensing [8] , indicating that the Western Congo Basin in Gabon and Southern Cameroon, and Eastern DRC support higher carbon stocks. We attribute this low stock mainly to a difference in diameter–height relationships. The lower carbon stocks and reduced canopy height at YGB could be related to climate and soil properties, the local available species pool or past natural and anthropogenic disturbances [8] , [18] , [19] , [20] , [21] . Disturbances due to past selective logging can have a substantial impact on forest structure [22] and, therefore, on carbon stocks. Nevertheless, based on our own field observations, analysis of the species composition ( Supplementary Fig. S1 ), communication with local foresters and an assessment of historical archives of the YGB station, we found no single indication that selective logging activities have been conducted in the study area in the last 150 years. Disturbance due to edge effects [23] , [24] could be a factor for some plots close to the edge ( Supplementary Fig. S2 ), but this effect remains negligible as we did not observe a significant difference between these plots and the plots at a longer distance from the edge. Relatively high average air temperatures in this lowland study area could explain the lower standing biomass because it may cause increased turnover rates and photosynthetic inhibition [25] . This could be an important factor, but in itself cannot explain the significantly lower carbon stock in YGB as the mean annual temperatures in Ituri and Dja are similar to that in YGB. The effect of soil conditions is probably more important here. Soils in our study area are sandier compared to those in Dja and Ituri ( Table 2 ), with sandy soils generally characterized by lower fertility and more limited water retention. The low N content and the high sand fraction in YGB indicate resource-poor soils, both in terms of nutrients and water availability. This low N content is also found in Dja and Ituri, but the sand fraction in these soils is lower providing a higher water holding capacity, specifically in Dja. Additionally, the higher bulk density for the more sandy soils in YGB indicates more compaction, which influences root penetration and reduces water infiltration. These soil properties can have an effect on height–diameter relationships [26] through nutrient limitations or a reduced water holding capacity, both of which influence the amount of carbon stored in biomass. In addition, there may be issues with mechanical instability in sandy soils [21] , increasing natural disturbances and leading to a lower standing biomass, or favouring smaller trees. This soil effect could be a driver for the differences in carbon stocks between YGB and Dja, with height–diameter relationships being the main structural difference between these sites, both for mixed and mono-dominant forests. A lower maximal tree height is reached on resource-poor and less stable soils in YGB. Also in the mono-dominant forests of Ituri, tree height is a major factor driving the higher biomass, but the comparison with mixed forests in Ituri highlights wood density as an additional factor. In these forests, a higher mean wood density is found compared with the YGB sites, with the Ituri sites on less sandy soils. In the study by Gourlet-Fleury et al. [5] the contrary was shown, with higher carbon stocks in less fertile regions due to a tendency to support slow-growing species with a higher wood density and possibly due to a slower turnover rate [27] . Nevertheless, we show that when eliminating differences in the species pool, via the analysis of mono-dominant forests, a lower aboveground carbon stock on less fertile soils of YGB is explained through a lower maximal tree height. To date, no clear general relationship has been established between forest carbon stocks and soil properties, and the available results are contradictory [5] , [18] , [21] , [28] . If soil texture or other soil properties are indeed related to forest structure, applying equations developed from trees on a different soil type could give rise to highly inaccurate carbon stock estimates across the Congo Basin. Regressions based on large subcontinental regions that are used [14] , [17] , may need to be replaced with a regional approach or an approach based on climatic or soil classifications. However, the spatial distributions of soil type, forest structure and carbon stocks in tropical Africa are poorly known [8] , [29] and quantification of the carbon emission and storage potential of these forests remains challenging. At local scales, emissions resulting from deforestation, degradation and regrowth can be determined by measuring forests at different stages of degradation [6] . Looking at different regrowth stages in our study area, we made two main observations. First, within the first few decades of regrowth, the aboveground carbon stock did not return to its initial state. This trend could persist, as tree species composition has changed and there is a tendency towards species with a lower wood density ( Supplementary Table S2 ), hence decreasing the total carbon stock of this type of disturbed forest. Secondly, soil carbon stocks remain high even after degradation of the forest ( Fig. 4 ), but do show sensitivity to land-use change. An initial nonsignificant soil carbon decline is observed due to forest clearing for agricultural use. However, the stock rapidly increases to a significantly higher level after two decades of regrowth. Because of the large amount of carbon stored in the soil it will be crucial to quantify the impact of possible future agricultural intensification, as land use after deforestation has significant potential effects on soil carbon [30] , [31] , [32] . If future demand for agricultural crops exceeds the yield of the traditional agricultural activities, agricultural intensification will become a necessity. This intensification could eventually require less land than currently to sustain the local population [33] , [34] , thereby securing the remaining forest and its carbon stock. However, the choice of agricultural system will critically affect the carbon balance. Land management can, depending on the disturbance intensity, drastically change the amount of carbon stored in the soil, with tillage and fertilization affecting soil disturbance and carbon decomposition rates [30] . The local integrated carbon balance of different agricultural systems therefore needs to be considered. In the context of climate change mitigation policies (for example, REDD) for tropical Africa, major challenges remain. Our results show that height–diameter regressions developed from data obtained from forest sites in the outer regions of the Congo Basin do not produce accurate aboveground carbon stock estimates for central areas of the basin. The current best carbon stock estimate for structurally intact closed canopy African tropical forest [11] of 202 Mg C ha −1 is, therefore, probably an overestimate. There are significant consequences of the 24% overestimation of aboveground carbon stocks in YGB. With annual net deforestation and degradation rates in the Congo Basin estimated to be 0.17% and 0.09%, respectively, between 2000 and 2005 (ref. 35 ), this biased carbon stock estimate could result in an overestimation of carbon loss. Nevertheless, confirmation of our results is needed through the establishment of inventory plots throughout the basin covering a larger area. Allometric equations developed specifically for Central Africa and pan-tropical models need to be validated and updated to improve the quality of regional and national carbon stock inventories. In addition, the spatial distribution, variability and response to future climate of soil carbon stocks are practically unknown [29] , [31] . We conclude that a spatially explicit understanding of both the aboveground carbon and the soil carbon stock remains crucial in developing an overall carbon budget for tropical African forests in order to support current and future climate policy measures. Study area This study was carried out in the UNESCO Man and Biosphere reserve in YGB, ~100 km west of Kisangani, DRC. The reserve covers an area of 6,297 km 2 (ref. 36 ), just north of the Congo River, and all study sites are located in the south-western (N00°47′; E24°30′) and north-western part (N00°59′; E24°32′) of the reserve. The region has an Af-type tropical rainforest climate [37] (following Köppen–Geiger). The site receives upto 1,762±295 mm per year (1961–2010) of rain and has one dry season from January to February with monthly precipitation lower than 100 mm (ref. 50 ). Temperatures are high and constant throughout the year with a minimum of 24.2±0.4 °C in July and a maximum of 25.5±0.6 °C in March. Soils in the YGB plateau are ferralsols primarily formed from aeolian sediments, composed mostly of quartz sand, kaolinite clay and hydrated iron oxides [38] , [39] . Vegetation in the reserve is characterized by moist semideciduous rainforest, with fragments of moist evergreen rainforest, transition forest, agricultural land, fallow land and swamp forest [38] . Plot selection and inventory A preliminary classification of the study area was made using SPOT-4 HRVIR, Landsat and geo-eye satellite images [40] using an object based classification approach. Plot locations were assigned within each classification type before fieldwork. The forest type was validated in the field and permanent inventory plots of 1 ha have been installed [41] , [42] . Topography of the region is gentle, and squared or rectangular plots were realized on the ground (no projected area). A standardized international inventory protocol for tropical forest was used [42] (RAINFOR) to assure comparability with other studies. All live stems with a diameter larger than 10 cm were tagged, measured for diameter at breast height at 1.3 m and identified upto species level. Buttressed trees, although a rarity in the region, and stilt-rooted trees are measured 50 cm above the highest root, where the trunk shape is cylindrical. When a deformity is present at breast height, the diameter is measured 2 cm lower. Species identification was done with the help of local botanists of the Institut National pour l’Etude et la Recherche Agronomiques. Height measurements All tree individuals were classified in the field into diameter classes (that is, 10–20, 20–30, 30–50, >50 cm) and all species contributing to 95% of the basal area of the plot were selected for further measurement. For each of these species, two individuals were selected within each diameter class. These individuals were measured for tree height using a Nikon Laser Rangefinder Forestry Pro hypsometer. The top of the tree is determined from different view angles and multiple measurements are made to account for over- or underestimation. When the top of an individual is not visible, a different individual using the same selection criteria is selected. Wood density measurements The same individuals selected for tree height measurements are selected for wood sampling to determine species wood density, defined as the ratio of oven dry weight and fresh volume. Wood samples with an average size of 5 × 5 × 5 cm 3 are taken under the bark. For those species with no wood density data, a genus-average was taken or when genus data was unavailable, a family-average was used. For a few remaining species from which the family did not occur elsewhere in the plot and for the remaining unidentified individuals, a site-average was used. Mean wood density for each plot was weighted by basal area. Height–diameter regressions Stand-specific height–diameter regression models were developed for each forest type. All trees known to be broken, damaged or leaning more than 10% were excluded from the analysis. Weibull, Chapman–Richards, logistic, power and two- and three-parameter exponential models were compared. The optimal model was selected based on the Akaike Information Criterion and the residual standard error, and was further used to determine tree heights for aboveground carbon stock estimation. No tree height measurements are available for old regrowth forest ( n =1), and the model for mixed semideciduous forest was used as similar species were present. Allometric equations The relation of Chave et al. [13] for moist tropical forest including height and wood density was selected for aboveground carbon stock estimation, with biomass assumed to be 50% carbon. Soil carbon storage Soil cores were collected using five depth increments: 0–10, 10–20, 20–30, 30–50 and 50–100 cm. From each replicated plot per forest type a composite soil sample ( n =10) was prepared per depth. Composite samples were oven-dried at 50 °C. Carbon content was determined via element analyses using continuous flow EA-IRMS. For each depth increment, carbon stocks (Mg C ha −1 ) were determined as a product of bulk density (g cm −3 ), carbon concentration (%) and thickness of the increment layer (cm). Soil texture was determined by means of the percentage of sand, silt and clay. Analyses were performed on air-dried soil fractions (<2 mm). The sand fraction (>63 μm) was separated by wet sieving; the silt and clay fractions were determined by the pipette method of Köhn after dispersion with sodium hexametaphosphate [43] . Statistics One-way analysis of variance is used followed by a Tukey honestly significant difference test to compare the means of the AfriTRON sites [11] and the YGB sites. To compare the carbon stocks of the different forest types in YGB, Fisher’s least significance difference test is used. How to cite this article: Kearsley, E. et al. Conventional tree height–diameter relationships significantly overestimate aboveground carbon stocks in the Central Congo Basin. Nat. Commun. 4:2269 doi: 10.1038/ncomms3269 (2013).